Helicity-dependent single-walled carbon nanotube alignment on graphite for helical angle and handedness recognition Aligned single-walled carbon nanotube arrays provide a great potential for the carbon-based nanodevices and circuit integration. Aligning single-walled carbon nanotubes with selected helicities and identifying their helical structures remain a daunting issue. The widely used gas-directed and surface-directed growth modes generally suffer the drawbacks of mixed and unknown helicities of the aligned single-walled carbon nanotubes. Here we develop a rational approach to anchor the single-walled carbon nanotubes on graphite surfaces, on which the orientation of each single-walled carbon nanotube sensitively depends on its helical angle and handedness. This approach can be exploited to conveniently measure both the helical angle and handedness of the single-walled carbon nanotube simultaneously at a low cost. In addition, by combining with the resonant Raman spectroscopy, the (n,m) index of anchored single-walled carbon nanotube can be further determined from the ( d , θ ) plot, and the assigned (n,m) values by this approach are validated by both the electronic transition energy E ii measurement and nanodevice application. Single-walled carbon nanotubes (SWNTs) have been regarded as promising building blocks for future nanoelectronic devices, because of their superb properties, including high carrier mobility, ideal subthreshold characteristic and large current-carrying capacity [1] , [2] . Horizontally aligned SWNTs are greatly desired for the integration of single SWNT devices into scalable integrated circuits [3] , [4] , [5] , [6] , [7] . As the electronic properties of the SWNT sensitively depend on the precise assembly of C atoms in the tube wall or the SWNT helicity, the preparation of aligned SWNTs with selected or identified helicities is essential to achieve the optimum performance of the SWNT devices or circuits. Recently, the gas flow-directed and/or anisotropic substrate surface-directed growth modes have been exploited to align the SWNTs during their growth, but technologies that can be used to control or measure the helicities of these SWNTs are not available [8] , [9] , [10] , [11] . In the case of the anisotropic surface-mediated growth of SWNT arrays, the orientation of SWNTs is determined by the surface lattice or the atomic terraces on the high anisotropy substrate [12] , [13] . For example, SWNTs tend to be anchored along some specific orientations with a few commensurate angle increments of 60 o , 90 o and 120 o on the layered mica, MgO (001) and quartz (001) surfaces, respectively [12] . In this work, we develop an approach to produce the aligned SWNTs with recognized helical angles and handednesses on graphite, where the orientation of a SWNT is determined by both the helicity of the SWNT and the anisotropy of the graphite surface. This approach allows us to measure both the helical angles and handednesses of large numbers of anchored SWNTs in a simple and cheap manner. Moreover, by combining with resonant Raman spectroscopy, the (n,m) index of SWNT can be accurately determined from the ( d ,θ) plot for the nanodevice application. Theoretical calculations of the anchored SWNTs on graphite A SWNT, such as the (10,0), (7,2)-R, (5,5) or (2,7)-L (where R and L represent the zigzag right and left handednesses, respectively) [14] SWNTs shown in Fig. 1a , could be conceptually described as a hollow cylinder of a rolled-up graphene sheet (indicated by the rectangle). The wrapping vector (n,m) fully determines the diameter, helical angle and handedness of the SWNT. The (7,2)-R and (2,7)-L are the enantiomers [15] with a relationship of θ (7,2) + θ (2,7) =60°, where θ is the helical angle of the SWNT. The van der Waals interaction between two graphite layers is strongest when their configuration is AB stacking. Similarly, the maximum interaction between a SWNT and graphite can be achieved if their interface has the similar AB stacking geometry ( Fig. 1b–e ) [16] , [17] , [18] . As such, the zigzag (10,0), chiral (7,2)-R and (2,7)-L and armchair (5,5) SWNTs prefer to be anchored along the perpendicular directions of the 0°+ i × 60°, 12.2°+ i × 60°, 47.8°+ i × 60° and 30 o + i × 60° on graphite, respectively (where i is an integer), as indicated by the red solid lines in Fig. 1a . In this way, the graphite has overwhelming advantages as a substrate to align SWNTs for both helical angle and handedness recognition. 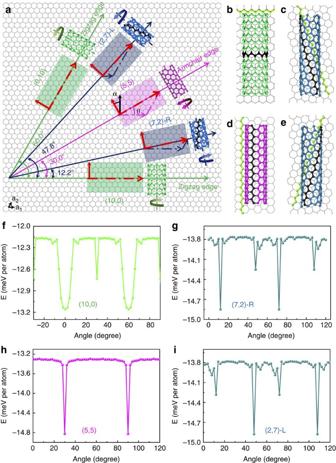Figure 1: Helicity-selective alignment of SWNTs on a graphite surface. (a) The zigzag (10,0) and (0,10), armchair (5,5), and chiral (7,2)-R and (2,7)-L SWNTs can be obtained by rolling up graphene sheets (rectangles with different colours) along their wrapping vector directions. The red dash–dot and solid lines indicate the wrapping vectors and tube axes, respectively. The top views of the SWNT–graphene interfaces are shown inb–e, where only the interfacial parts of SWNTs are shown. The interaction energies between SWNTs and their underlying graphene for (10,0), (7,2)-R, (5,5) and (2,7)-L SWNTs are shown inf–i, respectively. Figure 1: Helicity-selective alignment of SWNTs on a graphite surface. ( a ) The zigzag (10,0) and (0,10), armchair (5,5), and chiral (7,2)-R and (2,7)-L SWNTs can be obtained by rolling up graphene sheets (rectangles with different colours) along their wrapping vector directions. The red dash–dot and solid lines indicate the wrapping vectors and tube axes, respectively. The top views of the SWNT–graphene interfaces are shown in b – e , where only the interfacial parts of SWNTs are shown. The interaction energies between SWNTs and their underlying graphene for (10,0), (7,2)-R, (5,5) and (2,7)-L SWNTs are shown in f – i , respectively. Full size image To confirm the above analysis, theoretical calculations based on the registry-dependent interlayer potential [19] were performed to explore the interfacial energies between SWNTs and the graphite surface (see Methods for more details). In agreement with previous analysis, the results in Fig. 1f–i clearly show that the (10,0), (7,2)-R, (5,5) and (2,7)-L SWNTs have sharp minima precisely at 0°+ i × 60°, 12.2°+ i × 60°, 30°+ i × 60° and 47.8 o + i × 60°, respectively. The small peak in the potential energy surface is a consequence of the ‘pseudocommensuration’, which can be regarded as a geometric feature produced by the finite transverse extent of SWNTs. All the obtained angles have a periodicity of 60 o , which reflects the D 6h symmetry of the underlying graphene lattice. Growth and characterization of the anchored SWNTs To experimentally investigate the helicity selective alignment of SWNTs, the kite-flying process was used to grow SWNTs on the graphite surface ( Supplementary Figs S1 and S2 ). The atomic force microscopy (AFM) images shown in Fig. 2a,b clearly indicate that each SWNT tends to be anchored along a few directions and the alignment angle differences are 180 o , 120° or 60°, which indicates the equivalence of these orientations due to the D 6h symmetry of the graphene lattice. To identify the orientation of these aligned SWNTs, catalytically etched trenches along zigzag directions are used to mark the crystallinity of the graphite ( Supplementary Fig. S3 ) [20] , [21] . The angles between the two SWNTs and graphite trench are 69.8 o ( Fig. 2a ) and 45.7 o ( Fig. 2b ), respectively, and the angle between two anchored SWNTs on a same graphite surface is 18.5 o . All of these angles can’t be explained by the D 6h symmetry of graphene lattice and thus indicate that the SWNT alignment on the graphite surface is helical angle dependent. 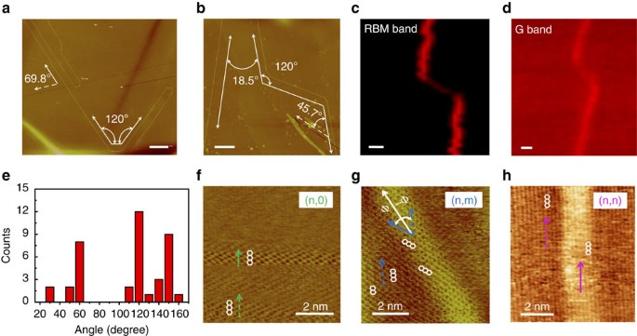Figure 2: Structure characterizations of the anchored SWNTs grown on graphite. (a) The typical AFM image of a self-organized SWNT with a turning angle of 120° and an angle of 69.8ofrom the etched trench on a graphite surface. (b) Two anchored SWNTs grown from13C-labelled CH4(one is straight and the other one changes its orientation twice). (c,d) Raman mapping results with radial breathing mode (c) and G (d) bands of the turned SWNT inb. Scale bars ina–d, 1 μm. (e) Histograms of turning angles of the grown SWNTs. (f–h) Atomically resolved STM images of the zigzag (f), chiral (g) and armchair (h) SWNTs on graphite surface. The arrows indicate the benzene ring arrangements (along zigzag edge) of SWNT upper parts (solid lines) and the graphite surface (dot lines). Figure 2: Structure characterizations of the anchored SWNTs grown on graphite. ( a ) The typical AFM image of a self-organized SWNT with a turning angle of 120° and an angle of 69.8 o from the etched trench on a graphite surface. ( b ) Two anchored SWNTs grown from 13 C-labelled CH 4 (one is straight and the other one changes its orientation twice). ( c , d ) Raman mapping results with radial breathing mode ( c ) and G ( d ) bands of the turned SWNT in b . Scale bars in a – d , 1 μm. ( e ) Histograms of turning angles of the grown SWNTs. ( f – h ) Atomically resolved STM images of the zigzag ( f ), chiral ( g ) and armchair ( h ) SWNTs on graphite surface. The arrows indicate the benzene ring arrangements (along zigzag edge) of SWNT upper parts (solid lines) and the graphite surface (dot lines). Full size image To further confirm that the produced linear structures observed by AFM were SWNTs rather than the possible wrinkles on the graphite surface, the 13 C-labelled CH 4 was used as carbon source to grow SWNTs on 12 C graphite. Both Raman images of RBM (radial breathing mode) band at 154.8 cm −1 and G band at 1,528.9 cm −1 ( Fig. 2c,d ) displayed the same turning orientation with the turned SWNT in Fig. 2b and the excitation laser was 632.8 nm. Meanwhile, the G band of this SWNT had an obvious red shift compared with that of graphite ( Supplementary Fig. S4 ) [22] . Therefore, we confirmed that the produced linear structures were the grown SWNT. Furthermore, a histogram of the turning angles, measured by AFM images of the turned SWNTs, showed three high peaks at 120 o , 150 o and 60 o ( Fig. 2e ). All the evidence clearly indicate that the alignment of the SWNTs on graphite is helicity dependent and, thus, is different from that on previously used surfaces, such as SiO 2 , quartz and sapphire. Scanning tunnelling microscopy (STM) characterizations [23] , [24] were performed to explore the atomic structures of SWNTs on the graphite ( Supplementary Figs S5–S6 ). As described above, the SWNT–graphite interaction is dominated by the interfacial structures of the SWNT and graphite, whereas only the upper surface of the SWNT can be characterized by the STM. Hence, it is necessary to construct their interface configurations from the STM images. As we know, both the achiral zigzag and armchair SWNTs have the same benzene ring arrangements (the arrangement is defined along zigzag edge) at the upper and lower surfaces of the SWNT from the top views ( Fig. 1b,d ). For chiral SWNT, the benzene ring arrangements at the upper and lower surfaces are different and are determined by a rotational symmetry as shown in the Fig. 2g (Φ is the angle between the SWNT axis and the zigzag edge of benzene ring arrangements). Although it is difficult to extract the (n,m) index of a SWNT directly from these STM images, the relative benzene ring arrangements of each SWNT and that of underlying graphite could be obtained by optimizing the scanning conditions. Figure 2f,h are the STM images of a zigzag (scanning direction parallel to the tube axis) and an armchair SWNT on graphite substrates, whose benzene ring arrangements are simultaneously shown. For both cases, the benzene ring arrangements in the SWNTs and the graphite are perfectly in agreement with each other, indicating the helical angle dependent alignment of zigzag and armchair SWNTs on graphite. Figure 2g is a STM image of a chiral SWNT with Φ=26.6°, and thus the direction of benzene ring arrangement of its lower surface should be Φ=−26.6° from the tube axis. As expected, the benzene ring arrangements of SWNT’s lower part are along the exact crystallinity orientation of the graphite substrate. Therefore, here we firmly proved that the alignment of a SWNT on graphite is helicity-selective. Helical angle and handedness determination of the SWNTs The ability to simply and fully characterize the helical structures of SWNTs, including both helical angle and handedness, has remained elusive despite much effort [25] . To the best of our knowledge, there is still lack of practical methods to characterize the chiral handedness of SWNTs besides the challenging techniques, such as STM and high-resolution transmission electron microscopy. Other characterization procedures, such as ultraviolet-visible and photoluminescence spectroscopy are not well suitable for the measurement of single SWNT, and the Raman spectroscopy [26] and Rayleigh scattering [27] are generally limited by the environment effect or resonance window. It is therefore extremely important to develop a simple and practical method to characterize the helical angle and handedness of SWNTs. Determining the benzene ring arrangements of a SWNT is crucial to recognize its helical angle and handedness [28] . As described above, the stable configuration of an SWNT on graphite surface tends to be anchored along the perpendicular direction to its wrapping vector. By taking the graphite zigzag edge as the reference [20] , the helical angle and handedness of each aligned SWNT can be easily characterized by AFM or STM imaging. From the AFM images, it is easy to obtain the angle ϕ (0 o < ϕ <60 o ) between the SWNT axis and the graphite zigzag direction marked by the etched trenches. If the measured ϕ ranges from 0 o to 30 o (red triangular area in Fig. 3a ), the SWNT is right handed and its helical angle is θ =30 o − ϕ . If the measured ϕ ranges from 30 o to 60 o (blue triangular area in Fig. 3a ), the SWNT is left handed and its helical angle is θ =90 o − ϕ . In this regard, the helical structure of a SWNT can be simply determined by AFM imaging. For example, in Fig. 3b , ϕ =83.7 o , which is equivalent to ϕ =83.7 o −60 o =23.7 o , owing to the graphene symmetrical lattices, so this SWNT is right handed with a helical angle of θ =30 o −23.7 o =6.3 o . In Fig. 3c , ϕ =39.6 o , so this SWNT is left handed with a helical angle of θ =90 o –39.6 o =50.4 o . 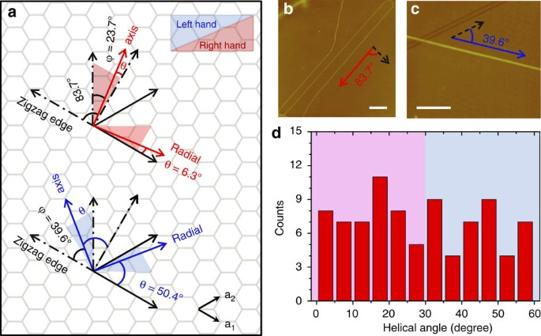Figure 3: Helical angle and handedness measurement of the SWNT on graphite surface. (a) Schematic diagram of measuring helical angles and handednesses of SWNTs. (b,c) AFM images of two SWNTs with angles of 83.7° (red triangular area ina) and 39.6° (blue triangular area ina) from the graphite trenches, respectively. Scale bars inbandc, 1 μm. (d) Histograms of helical angles and handednesses of 86 measured SWNTs. Figure 3: Helical angle and handedness measurement of the SWNT on graphite surface. ( a ) Schematic diagram of measuring helical angles and handednesses of SWNTs. ( b , c ) AFM images of two SWNTs with angles of 83.7° (red triangular area in a ) and 39.6° (blue triangular area in a ) from the graphite trenches, respectively. Scale bars in b and c , 1 μm. ( d ) Histograms of helical angles and handednesses of 86 measured SWNTs. Full size image Using this methodology, it is quick and easy to determine the helical structures of each SWNT in aligned arrays. The helical angle and handedness histogram of 86 SWNTs ( Fig. 3d ) indicates an equivalent possibility of a SWNT to be right handed and left handed, which means Fe catalysts with different sizes have the similar catalytic efficiency for SWNT enantiomers. In addition, we can clearly see that there is no obvious helical angle selectivity in the ultra-long SWNT sample. Moreover, the (n,m) index of each SWNT in arrays can be simply and uniquely determined by the ( d ,θ) plot ( Fig. 4a ), which can offer plenteous properties of SWNT, including the handedness (R or L) and conductivity (semiconducting (S) or metallic (M)). In Fig. 4b , the SWNT is right handed with a helical angle of 2.7 o . Its diameter can be calculated [26] by d =248.3/ ω RBM =248.3/169.8 cm −1 =1.46 nm. As thus, the (n,m) index of SWNT is (18,1)-R-S from the ( d , θ ) plot. Similarly, the SWNT in Fig. 4d is left handed with θ =33.4 o and d =1.96 nm. As thus, the (n,m) index of SWNT is (13,16)-L-M. To test the accuracy of the ( d ,θ) method, electronic transition energy E ii were obtained by the anti-Stokes/Stokes resonant Raman intensity ratio [29] ( Supplementary Fig. S7 ). The I as / I s values of 0.650 ( Fig. 4b ) and 2.497 ( Fig. 4d ) indicate the E ii of 2.407 eV and 2.413 eV, which correspond to the E 33 S =2.396 eV of (18,1)-R and E 22 M =2.404 eV of (13,16)-L, respectively (see Supplementary Note 1 ) [26] . Finally, the field effect transistor devices of these SWNTs were fabricated, and the transport properties that displayed the (18,1)-R SWNT was semiconducting with I on / I off of about 10 5 and the (13,16)-L SWNT was metallic. Also, SWNTs with different helicities can be effectively separated for the fabrication of helicity-dependent SWNT devices (see Supplementary Fig. S8 and Supplementary Note 2 ). 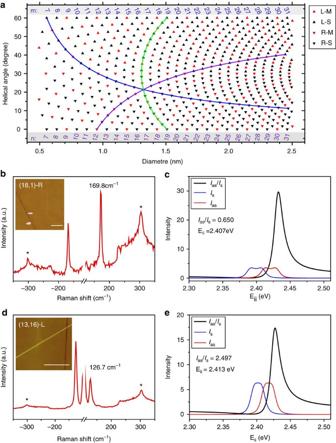Figure 4: Determination of chiral index of the anchored SWNTs. (a) The (d,θ) plot. The SWNTs have identical n, m and the sum of n and m in the violet, blue and green lines, respectively. R, L, M and S represent the right handed, left handed, metallic and semiconducting, respectively. (b), The anti-Stokes and Stokes Raman spectra of the inset SWNT and theωRBM=169.8 cm−1. (c)Ias/Isof the SWNT inbis plotted as theEii. (d) The anti-Stokes and Stokes Raman spectra of the inset SWNT and theωRBM=126.7 cm−1. The excitation laser energy is 2.41 eV. Scale bars of AFM images inbandd, 1 μm. (e)Ias/Isof the SWNT indis plotted as theEii. RBM, radial breathing mode. Figure 4: Determination of chiral index of the anchored SWNTs. ( a ) The ( d , θ ) plot. The SWNTs have identical n, m and the sum of n and m in the violet, blue and green lines, respectively. R, L, M and S represent the right handed, left handed, metallic and semiconducting, respectively. ( b ), The anti-Stokes and Stokes Raman spectra of the inset SWNT and the ω RBM =169.8 cm −1 . ( c ) I as / I s of the SWNT in b is plotted as the E ii . ( d ) The anti-Stokes and Stokes Raman spectra of the inset SWNT and the ω RBM =126.7 cm −1 . The excitation laser energy is 2.41 eV. Scale bars of AFM images in b and d , 1 μm. ( e ) I as / I s of the SWNT in d is plotted as the E ii . RBM, radial breathing mode. Full size image In summary, we have developed an approach to determine both the helical angle and handedness of SWNTs grown on graphite. It is proven that the alignment of SWNT on graphite was determined by both the SWNT helicity and the anisotropy of graphite surface. This approach was used to measure the helical angles and handednesses of SWNTs at a low cost. By combining with the resonant Raman spectroscopy, the (n,m) indices of the anchored SWNTs can be further determined from the ( d ,θ) plot. We believe that this approach has a great prospect for the future carbon-based nanoelectronics. Theoretical calculations In this calculation (see Supplementary Note 3 ), both the aligned SWNTs and graphite substrate are considered to be rigid and only a single rigid graphene layer was used to model the graphite, because the interaction between the SWNT and other graphene layers is negligible (the calculated error is less than 1%). The rotation angle α is defined as the angle between the tube axis and one armchair crystallinity orientation of the graphene lattice, which corresponds to the tube helical angle θ ( Fig. 1a ). In the calculation, we hold the rotation angle α fixed and optimize other freedoms of the SWNT (one rotation and three translations). Finally, the optimized interaction energy E (meV per atom) as a function of the rotation angle α was obtained. Growth of SWNTs The kite-flying process was used to grow SWNTs in a chemical vapour deposition system [30] . Few-layer graphene or graphite was mechanically exfoliated from the bulk Kish graphite (Covalent Materials Corp.) on Si substrates (300 nm oxide layer) by Scotch tape [31] . The FeCl 3 /EtOH solution was patterned on the other SiO 2 substrate as growth catalyst, which was predeposited near the graphite/SiO 2 substrate ( Supplementary Fig. S1 ). Then the substrates were placed in the quartz tube (1 inch) for SWNT growth. The chemical vapour deposition furnace was heated to 950 °C within 30 min by introducing 100 sccm Ar and 300 sccm H 2 . When the growth temperature reached, the EtOH vapour was used as the carbon source through a bubbler with 100 sccm Ar. After a period of 20 min, the EtOH vapour was turned off and the temperature was decreased from 950 o C to 850 o C within 1 h. Finally, the furnace was cooled to room temperature. The grown SWNTs and graphite were characterized by scanning electron microscopy (Hitachi S4800), AFM (Nanoscope IIIa) and Raman spectroscopy (Horiba HR800, with laser excitation at 632.8 nm and 514.5 nm). STM characterization of SWNTs The preparation process for STM sample and STM images of the graphite are shown in Supplementary Figs S5 and S6 , respectively. Before the STM characterization, the SWNT sample was annealed in flowing H 2 /Ar at 350 o C for 3 h to remove resist residues. Constant-current STM images were obtained with an Omicron ultra-high vacuum STM (tungsten tip, Fig. 2h and Supplementary Fig. S3c,d and e ) [28] and Nanoscope IIIa instrument (Pt-Ir tip, all other STM images) [24] at room temperature. The STM results strongly depend on the tip quality and scanning conditions ( Fig. 2f (610.0 mV and 518.0 pA), 2 g (438.6 mV and 229.4 pA) and 2 h (460.0 mV and 180.0 pA) were obtained under optimum scanning conditions). How to cite this article: Chen, Y. et al. Helicity-dependent single-walled carbon nanotube alignment on graphite for helical angle and handedness recognition. Nat. Commun. 4:2205 doi: 10.1038/ncomms3205 (2013).